Evidence of global-scale aeolian dispersal and endemism in isolated geothermal microbial communities of Antarctica New evidence in aerobiology challenges the assumption that geographical isolation is an effective barrier to microbial transport. However, given the uncertainty with which aerobiological organisms are recruited into existing communities, the ultimate impact of microbial dispersal is difficult to assess. Here we use molecular genetic approaches to examine microbial communities inhabiting fumarolic soils on Mount Erebus, the southernmost geothermal site on Earth, to evaluate the ecological significance of global-scale microbial dispersal. There, hot, fumarolic soils provide an effective environmental filter to test the viability of organisms that have been distributed via aeolian transport over geological time. We find that cosmopolitan thermophiles dominate the surface, whereas endemic Archaea and members of poorly understood Bacterial candidate divisions dominate the immediate subsurface. These results imply that aeolian processes readily disperse viable organisms globally, where they are incorporated into pre-existing complex communities of endemic and cosmopolitan taxa. Aeolian transport of microbes is the primary assumption inherent to Louren Baas Becking’s hypothesis that ‘everything is everywhere, but the environment selects’ [1] . Aerosolized microbes may originate from agricultural fields [2] , sewage treatment centres [3] , geothermal springs [4] , any surface exposed to sufficient wind force [5] and large-scale volcanic eruptions [6] . Organisms that have been independently aerosolized or attached to dust particles can be transported thousands of kilometres, which presumably allows microbes to easily move between continents and hemispheres [7] , [8] , [9] , [10] , [11] . The study of aerobiology is making great strides in showing that viable cells are attached to particles that are moved atmospherically [11] , [12] . However, these findings support only one of the two requirements for aeolian dispersal. While survival of cells on aeolian particles is necessary, successful dispersal of microorganisms also requires successful colonization of new habitats [13] . The presence of viable cells on actively transported particulates is therefore not sufficient to show that aeolian transport is capable of microbial dispersal. An ideal site for examining global-scale microbial dispersal would be one that is geographically isolated from similar sites and has habitat that is highly selective for viable organisms [13] . Mount Erebus, located on Ross Island in Victoria Land, Antarctica, fits these criteria extremely well [14] . It is the southernmost active volcano on Earth and possesses unique high-elevation geothermal features, such as ice caves and ice-free fumarolic ground that are located near its 3,794 m summit [15] . The geothermal features on Mount Erebus are separated from similar features on distant volcanoes by hundreds of kilometres of snow and ice, ensuring that locally sourced microbes are psychrophilic. The warm environments that are created by geothermal activity actively select against local psychrophiles, and encourage the growth of viable thermophiles and mesophiles that are endemic or have been sourced from distant features. The Tramway Ridge Antarctic Specially Protected Area (ASPA) ( Fig. 1a,b ), located ~1.5 km NW of the main crater of Erebus at an elevation between 3,350 and 3,400 m, is an extensive warm fumarolic area protected by international treaty as a site of particular biological interest (ASPA 130 Management Plan). It is located at the terminus of a lava flow that is ~10,000 years old and is composed primarily of phonolite, a fine-grained volcanic rock of alkali feldspars and nepheline [16] . A loose layer, as deep as 10 cm, of highly altered mineral soils lies atop the phonolitic base [15] . Within this ice-free area, small fumaroles emit steam and CO 2 , maintaining year-round average surface temperatures of 60–65 °C even during the coldest part of winter when air temperatures drop below −55 °C [17] . Subsurface concentrations of CO 2 and gas efflux rates vary considerably, even between fumaroles in close proximity [18] . Fumaroles are characterized by a neutral to mildly alkaline pH and are surrounded by steep lateral decreasing pH and temperature gradients that support unique assemblages of mosses and cyanobacterial mats [7] , [17] . 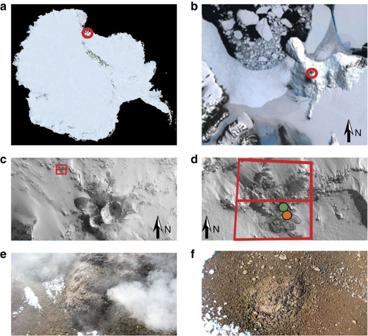Figure 1: Location of sampling sites in the present study. (a) Location of Ross Island in context of the continent of Antarctica. (b) Location of the summit of Mount Erebus in context of Ross Island. (c) View of the summit Caldera of Mount Erebus showing location of the Tramway Ridge Antarctica Specially Protected Area (ASPA) 130. (d) Location of sampling sites A (active fumarole-orange) and B (passive fumarole-green) within ASPA 130. Boundaries of the ASPA are denoted with red lines. Entry into the northern half of the ASPA is strictly prohibited. (e) Fumarole sampled as site A (active fumarole). (f) Fumarole sampled as site B (passive fumarole). Imagery provided by NASA LIMA (a), NASA Earth Observatory (b), Polar Geospatial Center © 2012 DigitalGlobe, Inc. (c,d), and S. Craig Cary (e,f). Figure 1: Location of sampling sites in the present study. ( a ) Location of Ross Island in context of the continent of Antarctica. ( b ) Location of the summit of Mount Erebus in context of Ross Island. ( c ) View of the summit Caldera of Mount Erebus showing location of the Tramway Ridge Antarctica Specially Protected Area (ASPA) 130. ( d ) Location of sampling sites A (active fumarole-orange) and B (passive fumarole-green) within ASPA 130. Boundaries of the ASPA are denoted with red lines. Entry into the northern half of the ASPA is strictly prohibited. ( e ) Fumarole sampled as site A (active fumarole). ( f ) Fumarole sampled as site B (passive fumarole). Imagery provided by NASA LIMA ( a ), NASA Earth Observatory ( b ), Polar Geospatial Center © 2012 DigitalGlobe, Inc. ( c , d ), and S. Craig Cary ( e , f ). Full size image A preliminary molecular community analysis of shallow (~2–4 cm depth) lateral transects showed that bacterial community structure varies significantly across much of the cool (<60 °C), low-pH (<7) expanse of Tramway Ridge; however, hot, neutral-pH steaming fumaroles share bacterial communities that are similar to one another [17] . The study showed that the fumaroles themselves are likely dominated by endemic taxa, including deep-branching Planctomycetes, Acidobacteria and Chloroflexi, as well as many novel, potentially division-level lineages with no known relatives [17] . The few Archaea observed at Tramway Ridge were all classified as Crenarchaeota and were most similar to environmental clones from subsurface environments in South Africa [19] and central Europe [20] . Here we examine the relevance of aeolian transport in the assembly of the microbial community inhabiting the fumarolic soils of Tramway Ridge. We characterize the composition of microbial communities with respect to depth within fumaroles at Tramway Ridge, determine which taxa are dominant and identify physicochemical factors that might structure communities within fumaroles. Vertical profiles were collected at two 65 °C fumaroles: one fumarole that vigorously emitted CO 2 and steam (active site, Fig. 1c ) and another that was visibly less active (passive site, Fig. 1d ). Amplicon pyrosequencing is used to assess community composition and structure within the soil profile at each fumarole, while shotgun DNA sequencing enables the reconstruction of full-length 16S rRNA genes that are used for high-resolution phylogenetic analysis. This survey reveals the co-occurrence of two distinct microbial communities, a surface community that is dominated by globally distributed populations and a subsurface community unique to Mount Erebus, demonstrating the importance of large-scale aeolian transport in the assembly of complex thermophilic communities. Physicochemistry Biologically relevant physicochemical parameters were measured for two soil profiles from Tramway Ridge ( Table 1 ) and limited variation between the active and passive fumaroles was observed: 65 °C at all sampling depths; 2.85–4.4% gravimetric water content; pH of 8.35–8.63; 64.7–81.6 μS conductivity; 0.20–0.44% total nitrogen; 0.12–0.62% total carbon. Subsurface oxygen concentrations revealed the subsurface atmosphere to be suboxic (~28% saturation) at each fumarole. While subtle, differences in physicochemistry were greater between samples taken from the active site (site A) than those from the passive site (site B) ( Supplementary Fig. 1 ) Table 1 Physicochemical data for the Tramway Ridge ASPA samples. Full size table Community structure of the Tramway Ridge ASPA fumaroles Microbial community structure was assessed by pyrosequencing multiplexed amplicons. 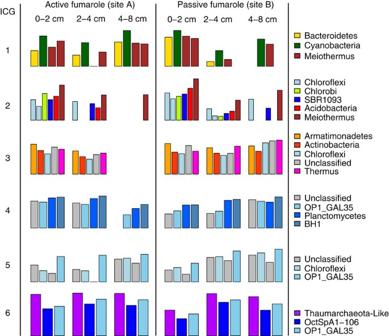Figure 2: Abundance profiles for 26 OTUs that were clustered into ICGs. ICGs are referred to in the text according to numeric designations in the far left column. Bar charts show the relative abundance of OTUs belonging to each ICG within each sample. Height of bars represents log-transformed relative abundance of each OTU in each sample. Theyaxis ranges from 5 × 10−5to 1 and is identical across samples and ICGs. Non-transformed relative abundances for each OTU may be found inSupplementary Table 1. In total, 111 operational taxonomic units (OTUs) were observed across all samples while the number of OTUs observed in any given sample ranged from 22 to 94 ( Table 2 ). As different numbers of sequences were generated across all samples, the read depth was normalized through bootstrap resampling to facilitate meaningful α-diversity and β-diversity calculations (see Methods). Pairwise dissimilarity indices were greater ( t -test P =0.051±0.004, N =3) within the vertical profile of the passive fumarole (average Morisita-horn dissimilarity=0.662; 95% CI: 0.197–0.957) than the more active fumarole (average Morisita-horn dissimilarity=0.069; 95% CI: 0.030–0.103) over all resamplings. The microbial community at both fumaroles had a marginally higher richness at the surface than in deeper substrata ( Table 2 ) and an inverse relationship was observed between the number of OTUs observed in a sample and sampling depth (Spearman ρ =−0.837, P =0.019, N =6). This relationship is consistent (bootstrap support) but weaker in resampled communities for both number of OTUs (Spearman ρ =−0.717, P =0.054, N =6, 95% CI: −0.717 -0.788, >99.9% bootstrap support for cor<0) and Chao1 diversity index (Spearman ρ =−0.717, P =0.054, N =6, 95% CI: −0.717–0.788, 99.8% bootstrap support for cor<0). Diversity metrics that include evenness were found to be less correlated with depth but showed consistency across resampled communities: ShannonH (Spearman ρ =−0.239, P =0.32, N =6, 95% CI: −0.239–0.120, >99.9% bootstrap support for cor<0); SimpsonsD (Spearman ρ =0.120, P =0.41, N =6, 95% CI: 0.120–0.120, 99.8% bootstrap support for cor>0). BEST analysis [21] failed to identify any physicochemical parameters that significantly describe variation in community structure using either Jaccard incidence distances (global P >0.10) or Morisita–Horn distances (global P >0.6). Table 2 Sequencing statistics and diversity metrics for total and resampled communities. Full size table Phylogenetic and thermal classification of fumarolic taxa The Tramway Ridge fumarolic community was found to be phylogenetically diverse, spanning 16 recognized Prokaryotic divisions, 8 candidate divisions and at least 5 unclassified lineages that conceivably represent novel divisions ( Fig. 2 , Supplementary Table 1 ). A few phyla such as Chloroflexi and Proteobacteria were well represented by large numbers of OTUs (10 and 16, respectively); however, they constitute vastly different portions of the community. Chloroflexi were present in all samples comprising up to 9% of all reads of a single amplicon library, while Proteobacteria was observed in only two samples and represent at most 1.1% of the reads in either. A single Archaeal OTU dominated the amplicon libraries, accounted for 40–60% of reads from each substratum at the active fumarole and showed much greater variation in samples from the passive fumarole (1.5–50.4%). Other prevalent taxa included Planctomycetes, Meiothermus, Cyanobacteria and members of the OP1_GAL35 and OctSpA1-106 lineages. Of the 111 OTUs that were observed at Tramway Ridge, 68 (61%) were found to be cosmopolitan and comprised between 32 and 92% of the summed relative abundances of any given sample. 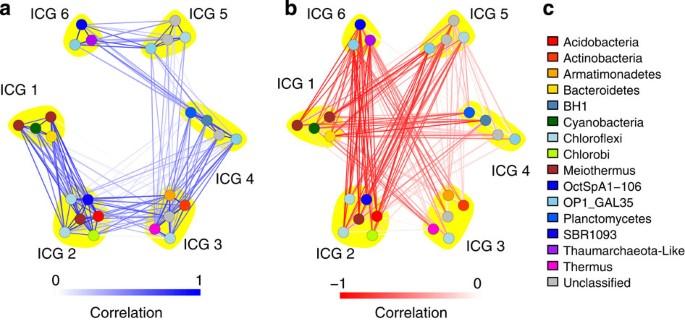Figure 3: Complete correlation network for twenty-six OTUs that clustered into ICGs. Nodes represent individual OTUs and are coloured by taxonomy. OTUs in each ICG are bound within a yellow area. (a) Blue lines represent positive correlation between OTUs. (b) Red lines indicate negative correlation between OTUs. The shade of lines are scaled according to strength of correlation as indicated by the colour key. (c) Colour key for taxonomic classifications. Cosmopolitan OTUs were further classified into one of five environmental categories based on the types of environment in which their non-Antarctic members have been observed ( Table 3 , Supplementary Table 1 , Supplementary Fig. 2 ). Almost 31% (34/111) of all OTUs were classified as non-thermal and made up 5–30% of the total number of OTUs observed in resampled communities ( Table 3 ). The surface (0–2 cm) sample from the passive fumarole in particular showed the greatest diversity of non-thermal taxa, with over 25% of all OTUs observed related to non-thermal lineages, collectively comprising 8.5% of the total reads in that sample. Over both profiles, the proportion of OTUs that were classified as non-thermal decreased marginally with depth (Spearman ρ =−0.717, P =0.054, N =6, 95% CI: −0.837 -0.478, 99.9% bootstrap support for cor<0) and the proportion of OTUs classified as thermal increased marginally with depth (Spearman ρ =0.717, N =6, P =0.054, 95% CI: 0.598–0.837, 99.9% bootstrap support for cor>0). Figure 2: Abundance profiles for 26 OTUs that were clustered into ICGs. ICGs are referred to in the text according to numeric designations in the far left column. Bar charts show the relative abundance of OTUs belonging to each ICG within each sample. Height of bars represents log-transformed relative abundance of each OTU in each sample. The y axis ranges from 5 × 10 −5 to 1 and is identical across samples and ICGs. Non-transformed relative abundances for each OTU may be found in Supplementary Table 1 . Full size image Table 3 Incidence of environmental classifications for each total and resampled data set. Full size table Networks reveal structured groups of organisms Microbial association network analysis was used to cluster OTUs into intra-correlated groups (ICGs). Network techniques are increasingly used in microbial ecology studies to infer ‘interactions’ between individuals in a community and indicate that taxa vary in a coordinated fashion across different samples [22] , [23] . The Benjamini–Hochberg procedure was used to estimate the false-discovery rate within our ICG analysis. A P -value cutoff of <0.001 created a ‘complete’ network of 33 OTUs connected by a total of 110 edges. This P -value cutoff corresponds to a false-discovery rate of 2.8% to 4.6%, suggesting that it included between 3 and 5 spurious connections. We also required that correlations be >0.8 to define an ICG, which removed 7 OTUs from our network, leaving behind 26 OTUs connected by 28 edges. Assuming that strong correlations (>0.8) are not particularly biased towards being spurious, we estimate that we may have retained one spurious false connection within our ICG-defining network. While a minority of the total diversity was captured in the six robust ICGs (26 OTUs), together these taxa account for 88–95% of all reads from any given sample ( Fig. 2 ). Positive correlation values below the ICG-defining threshold ( r >0.8) also reveal potential relationships among OTUs belonging to different ICGs ( Fig. 3a ). These potential connections were strongest between ICGs 1 and 2 (average r =0.600±0.162), between ICGs 3 and 4 (average r =0.577±0.108) and between ICGs 5 and 6 (average r =0.468±0.180). Negative correlations, which may either reflect an antagonistic or an independent relationship between sets of OTUs were also observed between the OTUs that comprise individual ICGs ( Fig. 3b ). Negative correlations were strongest between OTUs assigned to ICG 2 and those assigned to OTUs in ICG 6 ( r =−0.806±0.098). Figure 3: Complete correlation network for twenty-six OTUs that clustered into ICGs. Nodes represent individual OTUs and are coloured by taxonomy. OTUs in each ICG are bound within a yellow area. ( a ) Blue lines represent positive correlation between OTUs. ( b ) Red lines indicate negative correlation between OTUs. The shade of lines are scaled according to strength of correlation as indicated by the colour key. ( c ) Colour key for taxonomic classifications. Full size image Full-length rRNA gene analysis Twelve full-length 16S rRNA genes were reconstructed from shotgun sequencing of reads from bulk environmental DNA ( Supplementary Table 2 , Supplementary Fig. 3 ) and used for phylogenetic analysis ( Supplementary Fig. 4 ). These full-length sequences corresponded to the most abundant (>10% relative abundance in any library) amplicon-derived OTUs from each sample and collectively represented the majority of total amplicons from the passive site (54–82%) and the active site (78–88%). These full-length sequences were affiliated with cyanobacterium Mastigocladus laminosus , three distinct lineages of Meiothermus , two Acidobacterial lineages, a thermally restricted lineage of Armatimonadetes, three thermally restricted Candidate Division lineages (OctSpA106 (ref. 24 ), GAL15 (refs 25 , 26 ) and OP1_GAL35 (refs 25 , 27 , 28 ), as well as a novel Archaeal sequence. Two of the full-length sequences were examined in detail because they appear to represent lineages restricted to the Tramway Ridge ASPA. The first, belonging to a Planctomycete, closely matched the sequence from an earlier clone library from the Tramway Ridge ASPA [17] , but matched no other sequence in the NCBI or Greengenes databases with more than 89% nucleotide identity. This taxon groups within a clade of environmental clones (99.97% posterior support) as a sister lineage to the Gemmataceae (>99.99% posterior support) within the Gemmatales (97.8% posterior support) ( Fig. 4a ). A full-length sequence was also reconstructed for the novel, dominant Archaeon observed in the amplicon data set. This particular Archaeon was most closely related (94% identity) to a single clone (GI# 14028778) from a subterranean hot spring in Iceland [29] and shared no more than 87.1% identity to any other sequence in the NCBI database. Phylogenetic analysis of this full-length 16S rRNA gene grouped it with Crenarchaeota and Thaumarchaeota, specifically suggesting that it is a deep-branching relative of the Thaumarchaeota ( Fig. 4b ). This novel Archaeon evaded amplification in a previous study [17] , most likely due to mismatches in both forward and reverse primers. Archaeal sequences found in the previous study were present in the current study as rare taxa and phylogenetically affiliated with group 1.1b of the Thaumarchaeota ( Supplementary Table 1 and Supplementary Fig. 4 ). 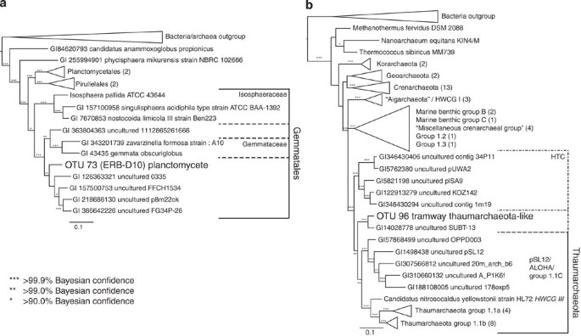Figure 4: Phylogenetic trees for full-length SSU-rRNA genes reconstructed from shotgun DNA sequencing. Trees are shown for the dominant Planctomycetes (a) and Archaeal (b) taxa found at the Tramway Ridge ASPA. Bipartitions were drawn at the 80% consensus level from a posterior distribution generated from 20 independent Markov chains. Bipartitions are designated as follows for posterior support: *90%; **99%; ***99.9%. Figure 4: Phylogenetic trees for full-length SSU-rRNA genes reconstructed from shotgun DNA sequencing. Trees are shown for the dominant Planctomycetes ( a ) and Archaeal ( b ) taxa found at the Tramway Ridge ASPA. Bipartitions were drawn at the 80% consensus level from a posterior distribution generated from 20 independent Markov chains. Bipartitions are designated as follows for posterior support: *90%; **99%; ***99.9%. Full size image Amplicon libraries of the 16S rRNA gene were used to examine the distribution of the geothermal microbial community in vertical profiles of fumaroles found on Mount Erebus. Two profiles were collected for analysis, one from an ‘active’ fumarole, vigorously emitting steam, and another from a ‘passive’ fumarole. Measured physicochemistry varied more at the active fumarole than at the passive fumarole ( Supplementary Fig. 1 ), yet the community structure showed greater stratification at the passive fumarole, as is evident from greater community dissimilarities observed in the depth profile. Subsurface oxygen measurements were similar between the two fumaroles and no additional physicochemical parameters (pH, conductivity, carbon, nitrogen, moisture, and so on) were identified to play a significant role in determining community structure. This suggests that currently unidentified soil physicochemistry variables, subsurface gas composition or other unknown characteristics may play a more significant role in determining the community structure within fumaroles than the variables measured in the current study. The microbial ecosystem of the Tramway Ridge ASPA fumaroles was dominated by an enigmatic relative of Thaumarchaeota, Aigarchaeota and Crenarchaeota ( Fig. 4b ) that showed very little sequence identity at the 16S rRNA gene level to other members of these groups (<89% identity). Similarly, a single lineage of Planctomycetes, nearly identical to a clone sequence previously reported for the Tramway Ridge ASPA [17] was identified as a deep-branching member of an uncultivated clade of mostly mesophilic members of the Gemmatales. In contrast, nearly all other dominant organisms were indistinguishable from cosmopolitan thermophiles that have been detected in neutral to alkaline terrestrial hot springs and associated sediments. These lineages include reasonably well-understood microbial mat taxa (Cyanobacteria and Meiothermus) as well as poorly understood divisions (Acidobacteria, OP1_GAL35, GAL15, OctSpA1-106 and Armatimonadetes). Mat-associated taxa, such as Cyanobacteria, were detected in the lowest substratum in both profiles. Given the proximity of Cyanobacterial mats to fumaroles, this was not surprising, yet it presented a challenge for identifying which taxa best represented thermophiles that were specifically associated with the fumarolic mineral soils. A microbial association network ( Fig. 3 ) based on correlation of relative abundance profiles was used to separate individual OTUs into structured subcommunities of dominant OTUs or ICGs. While compositional bias is a well-known problem when constructing correlation networks, we employed strategies that are believed to partially address these issues, such as the addition of pseudocounts and the use of in silico resampling procedures [30] . We further restricted our network definition of ICGs to include only those OTUs that are strongly ( r >0.8) correlated with one another. While these procedures have helped ameliorate falsepositive connections, they may have also fragmented our network by ignoring several true-positive connections. This may help explain why ICGs tend to comprise relatively abundant and well-represented OTUs and why pairwise correlations between OTUs belonging to specific pairs of ICGs are positively correlated with one another. Although only 26 out of 111 OTUs robustly clustered into 6 ICGs throughout multiple in silico resamplings, these OTUs nevertheless comprised 88–95% of amplicon reads from each sample ( Fig. 2 ) and enabled the separation of surface-associated taxa from the subsurface microbial community. Surface mat-associated subcommunities (ICGs 1 and 2) were dominated by Meiothermus sp. and Mastigocladus laminosus , the latter of which is known to dominate cyanobacterial mats at the Tramway Ridge ASPA [7] . The upper temperature limit for cultures of Tramway Ridge ASPA-specific strains of Mastigocladus laminosus is ~60 °C and at the Tramway Ridge ASPA, mats do not extend across the hot steaming fumaroles [7] , [31] , [32] . The presence of Mastigocladus laminosus in ICG 1 suggests that this subcommunity was restricted to cooler temperatures than 65 °C, the measured temperature of mineral soils at the time of sampling and the annual mean temperature previously reported for individual fumaroles at the Tramway Ridge ASPA [17] . Subcommunities defined by ICGs 1 and 2 include numerous additional lineages that are known to be associated with phototrophic microbial mats: Meiothermus sp., Bacteroidetes, Chlorobi and Chloroflexi. It is uncertain at this time whether the correlation of these taxonomic signatures with Cyanobacterial signatures indicates that these taxa were physically associated with fumarole-adjacent mats, or if it indicates that these taxa were inhabitants of the fumarole that were directly dependent on mat-derived materials. These subcommunities were proportionately greater in the surface (0–2 cm) of the highly stratified passive fumarole, and also included non-thermal OTUs ( Supplementary Table 1 ). Subsurface subcommunities (ICGs 5 and 6) were negatively correlated ( Fig. 3b ) with surface mat-associated subcommunities (ICGs 1 and 2). While it is important to keep in mind that increased abundances of one group of taxa will necessarily result in a decrease of another group of taxa when examining relative data, a negative correlation between two groups of taxa suggests independence, if not an antagonistic relationship. Therefore, we infer that OTUs in ICGs 5 and 6 are not likely to have been derived from surface mat-derived materials. We found that a novel relative of the Crenarchaeota, Thaumarchaeota and Aigarchaeota ( Figs 2 and 4 ) dominated the subsurface, as evidenced from amplicon library abundances and 16S reads from shotgun sequencing of environmental DNA. The exact relationship among the Aigarchaeota, hot Thaumarchaeota-related clade and Thaumarchaeota is currently being debated in the literature [33] , [34] , [35] and therefore phylogenetic analysis of a full-length reconstructed gene could not fully resolve whether this lineage should be included as a member of the Thaumarchaeota. Several demarcations are presented ( Fig. 4 ) that indicate robust monophyletic groupings with >99.0% posterior support and might provide reasonable phylogenetic limits to the Thaumarchaeota. In the present survey, we chose to refer to this lineage as Thaumarchaeota-like to capture this uncertainty and to differentiate between this relative of Thaumarchaeota and the recently described hot Thaumarchaeota-related clade lineages [35] , which forms its own, separate, well-supported clade. In addition the Thaumarchaeota-like taxon, subsurface subcommunities contained lineages of candidate divisions currently known only through 16S clone sequences. OctSpA1-106 was originally detected at Octopus Spring in Yellowstone National Park (USA) [24] and has since been detected at El Tatio Geyser Field (Chile) [36] , Uzon Caldera (Russia) [37] and terrestrial hot-spring areas in North America [28] , [38] . It has been detected only in neutral to alkaline, geothermally heated environments. The full-length 16S sequence from Tramway Ridge is 96% identical with the original type clone sequence (GI# 3800711) and 97% identical with clone GAL39 (GI# 84322458), both from Yellowstone National Park. The third lineage within ICG 6 is a member of Candidate Division OP1. However, the sequences in our data set are highly similar (98.55% nucleotide identity over the full-length 16S rRNA gene) to members of the GAL35 Class of Candidate Division OP1, and in our phylogenetic reconstructions ( Supplementary Fig. 4 ), this class forms a distinct division-level lineage, as has been observed by other researchers [28] . OTUs assigned to ICGs 3 and 4 were difficult to identify as either surface or subsurface-associated. The abundance of OTUs in ICGs 3 and 4 decrease with depth over the profile at the active site (site A), but are most abundant in the deepest substratum at the passive site (site B). OTUs assigned to these ICGs include novel lineages of Actinobacteria and Chloroflexi, as well as thermally restricted lineages of Armatimonadetes, Acidobacteria, Candidate Division BH1 and OP1 (GAL35). ICG 4 also included a novel lineage of Planctomycetes that was detected in an earlier study [17] and shown to be present in relatively high abundance in the current study. This full-length sequence could confidently be assigned to the Gemmatales (97.8% posterior support) ( Fig. 4a ) and potentially redefines the upper temperature limit for this Order at 60–65 °C. While the ‘Anammox’ lineages of Planctomycetes have been detected in high-temperature (>75 °C) environments [39] , the previous upper temperature limit for characterized members of the Gemmatales was ~55 °C ( Isosphaera pallida [40] ). We found that amplicons for the majority of OTUs (68/111) were highly similar (>97% sequence identity over 400 nt of the 16S rRNA gene) to clones reported from non-Antarctic environments ( Supplementary Table 1 and Supplementary Fig. 2 . These OTUs collectively accounted for 32–92% of the amplicons in any given sample library. As 16S rRNA is an inappropriate marker for distinguishing strains, our data was not used in an attempt to differentiate strain-level biogeography of species shared between Tramway Ridge and non-Antarctic environments. Nevertheless, within the resolution of our study, we propose that the ‘species’ represented by Tramway Ridge OTUs have likely been introduced to the Tramway Ridge ASPA through aeolian transport over the past several hundred thousand years. Aeolian dispersal has also been invoked to explain the incidence and movement of mat-associated Cyanobacteria, moss and algae among geothermal sites in Antarctica [7] , [31] , [41] , [42] . Atmospheric patterns suggest that South America is a likely source for Antarctic microbes. Over the glacial periods of the last 160,000 years, the majority of dust particles that were trapped in ice in Antarctica have been derived primarily from Patagonia [43] , [44] . Consistent with the aeolian input of mesophilic organisms into Antarctica, we found many non-thermal cosmopolitan OTUs at Tramway Ridge that were predominately found in the surface strata (0–2 cm) of both profiles. It is possible that these are signatures of organisms that have colonized the cooler areas adjacent to hot fumaroles and are distributed to fumarolic locations by the harsh winds at Tramway Ridge. Alternatively, some of these organisms may actually be living in a cooler, fumarolic surface crust that is too thin to detect within the resolution of our temperature probes (~1 cm). Regardless, the detection of diverse mesophilic cosmopolitan signatures at Tramay Ridge hints that the dispersal of organisms to the site may not be limited to thermophiles. Abundant, cosmopolitan thermophiles in our data set were classified as Mastigocladus laminosus , Meiothermus sp., Acidobacteria, OctSpA1-106 and OP1_GAL35 and are indistinguishable from those found in geothermal environments elsewhere. This suggests that each of these lineages possess adaptations for long-range dispersal. Interestingly, these OTUs match sequences from various areas known to be capable of ‘super-volcano’ scale eruptions, including the Yellowstone Caldera (USA) [24] , [27] , Altiplano-Puna Volcanic Complex (Chile, Bolivia) [36] and the Taupo Volcanic zone (New Zealand) [45] . Specific organisms, such as Mastigocladus laminosus , which form conspicuous microbial mats at the Tramway Ridge ASPA [7] , [17] have previously been hypothesized to have originated from Yellowstone Caldera and it has been suggested that they have subsequently become globally distributed through aeolian dispersal [46] . Our data set alone cannot be used to identify sources of the microbiota at Tramway Ridge, but volcanic events are readily detected in Antarctic ice cores and several of these can be traced to off-continent events [47] . While it remains difficult to understand how organisms might survive a typical pyroclastic eruption, a directed-blast explosion with enough force to eject material before superheating could potentially launch organisms and debris high into the atmosphere. Granted, the types of eruptions that might be capable of such an accomplishment would be large and rare, but it has been shown that even moderately large eruptions can disperse larger, eukaryotic organisms over vast distances [6] . Our results show that much of the diversity at Tramway Ridge is cosmopolitan and therefore that viable cells, from diverse divisions of the tree of life, are successful at global dispersal. While this ability is well known for particular Bacterial species [11] , [14] , [48] , [49] , [50] , others, especially thermophiles, are known to exhibit evidence of dispersal limitation [46] , [51] , [52] , [53] , [54] . Although these categorizations are largely dependent on temporal scaling [55] , our study did not examine potential strain-level endemicity of OTUs shared between Tramway Ridge and non-Antarctic sites, and all organisms probably exhibit some level of dispersal limitation [56] , here we have shown that global-scale dispersal nevertheless plays a significant role in the assembly of microbial communities over geological time periods. On the other hand, the presence of highly abundant, endemic populations suggests that specific organisms are uniquely adapted to this particular combination of environmental factors. These endemic taxa are defined explicitly by their ability to outcompete exogenous microbes, and their inability to disperse to other habitats. In our work, this principle is shown for thermophilic communities; however, there is no reason to suspect that this principle cannot be extended to mesophilic communities. We conclude that the process of microbial dispersal over global-scale distances must be considered as an important component of the general concept of microbial community assembly. Sample collection Sediment samples were collected within the Tramway Ridge Antarctic Specially Protected Area (ASPA 130) in February 2009 from two sites (site A (active site): 77° 31.103′ S, 167° 6.682′ S and site B (passive site): 77° 31.106′ S, 167° 6.668′ E). All suggested sterilization protocols for entering into this protected site were adhered to, following the ASPA 130 Management Plan ( http://www.scar.org/publications/bulletins/151/aspa130.html ). Sites were chosen based on measuring a surface temperature of 65 °C with a stainless steel Checktemp1 temperature probe (Hanna Instruments, Rhode Island, USA), sterilized with 70% ethanol immediately before each use. Surface ‘crust’ was set aside before collecting samples. Samples were collected by aseptically removing the top 2 cm of sediment in an ~25 cm 2 area. Sediment was placed into a fresh 50 ml Falcon tube. Sampling continued with the collection of a second (2–4 cm depth) and third (4–8 cm depth) layer following the same procedures. Temperature measurements were repeated for each layer sampled. All samples were immediately frozen, transported back to the University of Waikato frozen and maintained at −80 °C in the laboratory until analysed. Physicochemistry Samples were thawed and aliquots removed for pH/conductivity, total moisture content and carbon/nitrogen analyses. pH and conductivity was measured with the slurry technique, using 2 g of soil and 5 ml of deionized water, with a CyberScan PC 510 Bench Meter (Eutech Instruments Pte Ltd, Singapore). Water content was determined by drying 1 g of soil at 105C until a constant mass was reached over 3 consecutive daily measurements. For total carbon and nitrogen measurements, dried soil was ground to a fine powder using a ball grinder. Aliquots (0.2 g) were analysed using a LECO Truspec Elemental Determinator (LECO Corporation, St Joseph, MI, USA). Moisture content, pH, total carbon and total nitrogen were combined with previously collected physicochemistry data [17] and examined in a principal components analysis using the ‘rda’ function from the vegan package [57] in R (ref. 58 ). Subsurface fumarolic oxygen concentrations were measured in a subsequent trip to the Tramway Ridge ASPA (November 2011) using a Fibox 3 LCD trace minisensor oxygen metre (PreSens Precision sensing, Germany) that had calibrated for temperature and altitude at our base camp. DNA extraction, library preparation and sequencing DNA was extracted from samples using a modified CTAB (cetyltrimethylammonium bromide) bead-beating protocol [59] and quantified using the Quant-IT dsDNA HS Assay Kit (Invitrogen, Carlsbad, CA, USA). For shotgun sequencing, a portion of extracted genomic DNA was sequenced using standard protocols for the 454-Ti platform (Roche 454 Life Sciences, Branford, CT, USA) at the UCLA GenoSeq CORE. PCR amplicons containing V5–V7 hypervariable regions of the 16S rRNA gene were generated from the same genomic DNA samples using primers Tx9 (5′-GGATTA GAWACCCBGGTAGTC-3′) and 1391R (5′-GACGGGCRGTGWGTRCA-3′) [60] . PCR was performed in triplicate on each sample and pooled to reduce stochastic variation [61] . Three samples (site A 0–2 cm, site B 0–2 cm, site B 2–4 cm) were sequenced using the 454-GS-FLX platform by Taxon Biosciences (Tiburon, CA, USA) and three samples (site A 2–4 cm, site A 4–8 cm and site B 4–8 cm) were sequenced using the 454 Junior platform at the Waikato DNA Sequencing Facility (Hamilton, New Zealand). For the three samples sequenced using the 454-GS-FLX platform, each 30 μl reaction contained 2–10 ng of DNA extract, Pfx polymerase and platinum polymerase (0.5 U each; Invitrogen), 1 × Pfx PCR buffer with Pfx enhancer, 0.2 mM dNTPs, 1 mM MgCl 2 , 0.02 mg ml −1 BSA, 0.8 μM of forward and reverse primer and PCR-grade water. Thermal cycling conditions were 94 °C for 2 min; 24 cycles of 94 °C for 15 s, 55 °C for 30 s and 68 °C for 1 min; and 68 °C for 3 min. Amplicons were size-selected and purified using polyacrylamide gel electrophoresis before being prepared for pyrosequencing by Taxon Biosciences. For the three samples sequenced using the 454-junior platform, each 30 μl reaction contained 2–10 ng of DNA extract, PrimeStar polymerase (0.625 U; Takara), 1 × PCR buffer, 0.2 mM dNTPs, 0.4 μM of forward and reverse primer and PCR-grade water. Thermal cycling conditions were 94 °C for 3 min; 24 cycles of 94 °C for 20 s, 52 °C for 20 s and 72 °C for 45 s; and 72 °C for 3 min. Triplicate PCR reactions were pooled and gel-purified using the UltraCleanTM 15 DNA Purification Kit (MO BIO Laboratories Inc.), cleaned using the Agencourt AMPure XP Bead Cleanup kit (Beckman Coulter Inc.) and quantified (Quant-iTTM dsDNA HS Assay Kit, Invitrogen Ltd.). Cleaned amplicons were used as template (25 ng) in a second PCR reaction using fusion primers (forward: 5′-(454 Adapter A)-TCAG-MID-Tx9-3′; reverse: 5′-(454 Adapter B)-TCAG-1391R-3′). PCR conditions were exactly the same as the first round except only 10 cycles of PCR were performed. Triplicate PCR reactions were pooled and gel-purified using the UltraCleanTM 15 DNA Purification Kit, cleaned using the Agencourt AMPure XP Bead Cleanup kit and quantified (Quant-iTTM dsDNA HS Assay Kit) before being prepared for pyrosequencing using the 454 Junior platform by the University of Waikato sequencing facility. Sequence processing Shotgun sequencing reads were queried against a modified 16S rRNA gene database [62] using BLAST [63] . In all, 1,033 reads returned a bit score of >50 (see Supplementary Fig. 3 for histogram of all bit scores) and were assembled in Newbler (Roche 454 Life Sciences) using an overlap of 200 nt and per cent identity cutoff of 99% to produce near-full-length 16S rRNA genes. Near-full-length 16S rRNA gene sequences were aligned to 180 additional reference sequences using SINA [64] and the resulting alignment was used in a Bayesian phylogenetic analysis in Bali-Phy [65] with the following parameters: alignment=‘traditional’, iterations=11,000, burnin=6,000. Twenty independently seeded chains were initiated and independent posterior tree populations were pooled into a single posterior tree population from which consensus trees were built. 16S amplicon pyrosequencing results were processed using AmpliconNoise v1.22 to remove noise and filtered for chimeric reads using Perseus [66] . Reads were required to perfectly match MID sequences for processing. Sequence predictions from fewer than three individual raw reads or with at least one primer mismatch were discarded. Pairwise alignments/distances between sequence predictions were calculated using ESPRIT [67] and reads were clustered into OTUs using a distance cutoff of 0.03 and the average neighbour clustering algorithm ( Table 2 ) in Mothur [68] . OTUs that correspond to full-length sequences (>99% identity) were classified using our calculated phylogeny with a strict phylogenetic nesting criterion while remaining OTUs were classified taxonomically using classify.seqs in Mothur with 80% confidence as a threshold, using the Greengenes alignment and taxonomic outline released in November 2012 (ref. 69 ). Environmental classification of OTUs Each unique amplicon sequence was queried against the NCBI nr nucleotide database using BLAST [63] . Reads were classified as ‘thermal’ in the case that all database entries that matched the representative unique sequence with >97% identity had been previously observed in thermal environments, as ‘non-thermal’ if all matches were observed in non-thermal environments and as ‘polythermal’ if the matches were observed in a mixture of thermal and non-thermal environments. Reads for which the representative unique sequences only matched with <97% identity to any entries in the database were classified as ‘subnovel’ or ‘novel’ if the nearest match was between 95.5% and 97%, or <95.5%, respectively (see Supplementary Fig. 4 for histogram justifying these boundaries). Determination of ICGs OTUs were partitioned into ‘ICGs based on resampled correlation between relative abundance across all samples. First, ‘adjusted’ relative abundances were calculated by adding a single Bayesian pseudo-count to the number of counts observed for each OTU. This allowed every OTU to have a non-zero probability of occurrence in any sample. These revised counts were used as a probability vector to resample OTUs to the same depth (1,431 counts) within each sample using the sample() function in R (ref. 58 ). Resampling was carried out 2,000 times. For each resampling, Pearson correlations were calculated in a pairwise fashion between all OTU pairs using log-transformed relative abundances. OTU networks were constructed based on Pearson correlation coefficients exceeding 0.8 in >99.9% of resampled communities and visualized with R using the igraph package [70] . Sequence Data Accession: All raw data (*.sff files) for this study are available to the Sequence Read Archive as study number ERP002340 ( http://www.ebi.ac.uk/ena/data/view/ERP002340 ). Assembled near-full-length ribosomal RNA sequences are available at Genbank (Accession no. KF923316 - KF923327 ) How to cite this article: Herbold, C. W. et al. Evidence of global-scale aeolian dispersal and endemism in isolated geothermal microbial communities of Antarctica. Nat. Commun. 5:3875 doi: 10.1038/ncomms4875 (2014).